The key role of transient receptor potential melastatin-2 channels in amyloid-β-induced neurovascular dysfunction Alzheimer’s dementia is a devastating and incurable disease afflicting over 35 million people worldwide. Amyloid-β (Aβ), a key pathogenic factor in this disease, has potent cerebrovascular effects that contribute to brain dysfunction underlying dementia by limiting the delivery of oxygen and glucose to the working brain. However, the downstream pathways responsible for the vascular alterations remain unclear. Here we report that the cerebrovascular dysfunction induced by Aβ is mediated by DNA damage caused by vascular oxidative–nitrosative stress in cerebral endothelial cells, which, in turn, activates the DNA repair enzyme poly(ADP)-ribose polymerase. The resulting increase in ADP ribose opens transient receptor potential melastatin-2 (TRPM2) channels in endothelial cells leading to intracellular Ca 2+ overload and endothelial dysfunction. The findings provide evidence for a previously unrecognized mechanism by which Aβ impairs neurovascular regulation and suggest that TRPM2 channels are a potential therapeutic target to counteract cerebrovascular dysfunction in Alzheimer’s dementia and related pathologies. Alzheimer’s dementia (AD) has emerged as one of the major public health challenges of our times. Despite being a leading cause of death [1] , no disease-modifying treatment is available, and its impact will continue to grow, reaching epidemic proportions in the next several decades [2] . Accumulating evidence supports a role of cerebrovascular factors in the pathogenesis of AD [3] , [4] , [5] . Midlife vascular risk factors, such as hypertension, diabetes and obesity, increase the risk for AD later in life [6] , [7] . Autopsy studies have shown that mixed ischaemic and amyloid pathologies often coexist in the same brain, and that ischaemic lesions greatly amplify the negative impact of amyloid on cognition [8] , [9] . AD is associated with reductions in cerebral blood flow (CBF) early in the course of the disease [10] , [11] , [12] , as well as impairment of the ability of endothelial cells to regulate blood flow in systemic vessels [5] , [13] . In support of their pathogenic role, controlling vascular risk factors can slow down the progression of AD [14] and may have contributed to dampen the rise in AD prevalence [15] . Extracellular accumulation of amyloid-β (Aβ), a 40–42 amino-acid peptide derived from the amyloid precursor protein (APP), is a key pathogenic factor in AD. However, the mechanisms leading to the brain dysfunction underlying dementia remain to be fully established. In addition to its deleterious neuronal effects [16] , Aβ exerts potent actions on cerebral blood vessels [4] , [5] . Thus, Aβ 1–40 constricts blood vessels and impairs endothelial function, blood–brain barrier permeability and neurovascular coupling, a vital cerebrovascular response matching the increase in the energy demands imposed by neural activity with the delivery of substrates through CBF [17] , [18] , [19] , [20] . The mechanisms of the cerebrovascular effects involve activation of innate immunity receptors [21] , [22] , [23] , leading to the production of reactive oxygen species (ROS) by a NOX2-containing NADPH oxidase [24] , [25] . The cationic nonselective channel transient receptor potential melastatin-2 (TRPM2) is an important regulator of endothelial Ca 2+ homeostasis [26] , [27] . Thus, opening of the channel leads to a large Ca 2+ influx that has a deleterious impact on endothelial function and survival [28] , [29] . A defining feature of this channel is the presence of a C-terminus Nudix domain, which is responsible for its unique gating by (ADP)-ribose (ADPR) [28] , [30] . Aβ 1–40 leads to cerebrovascular accumulation of peroxynitrite, the reaction product of nitric oxide (NO) and superoxide [31] , [32] , which could induce DNA damage and activation of poly(ADP)-ribose polymerase (PARP) and poly(ADP)-ribose glycohydrolase (PARG) [32] . Since PARP/PARG activity is a major source of ADPR [32] , [33] , it is conceivable that Aβ-induced PARP/PARG activation in cerebral blood vessels leads to opening of potentially damaging endothelial TRPM2 channels. In the present study, we report that the endothelial dysfunction produced by Aβ 1–40 depends critically on nitrosative stress, PARP activity and TRPM2 channels, resulting in massive increases in intracellular Ca 2+ . The findings identify TRPM2 currents as a heretofore-unrecognized effector of Aβ 1–40 -induced endothelial vasomotor failure, and suggest that the TRPM2 channel is a putative therapeutic target for the neurovascular impairment associated with AD and related diseases. Peroxynitrite mediates Aβ-induced vasomotor dysfunction First, we sought to determine whether Aβ 1–40 induces nitration in the arterioles of the neocortical region in which CBF was studied, and, if so, whether such nitration contributes to the vasomotor dysfunction. Superfusion of the somatosensory cortex with Aβ 1–40 increased 3-nitrotyrosine (3-NT) immunoreactivity, a marker of peroxynitrite, in penetrating arterioles ( Fig. 1a ). The 3-NT increase was suppressed by the ROS scavenger Mn(III)tetrakis(4-benzoic acid)porphyrin Chloride (MnTBAP) or the NO synthase (NOS) inhibitor L-N G -Nitroarginine (L-NNA), and in NOX2-null mice ( Fig. 1b ), consistent with peroxynitrite being the source of the nitration. Aβ 1–40 also reduced resting CBF and attenuated the CBF increase produced by neural activity (whisker stimulation), by the endothelium-dependent vasodilator acetylcholine and the NO donor S-nitroso-N-acetylpenicillamine (SNAP; Fig. 1c ; Supplementary Fig. 1A ). Responses to adenosine and hypercapnia were not affected ( Fig. 1c ; Supplementary Fig. 1A ), attesting to the selectivity of the impairment of endothelial-dependent relaxation and neurovascular coupling. Next, we investigated whether peroxynitrite is involved in the vasomotor dysfunction. Neocortical application of the peroxynitrite scavenger uric acid (UA) or the peroxynitrite decomposition catalyst 5,10,15,20-Tetrakis(4-sulfonatophenyl)porphyrinato Iron (III), Chloride (FeTPPS), but not its inactive form TPPS, prevented the attenuation in the cerebrovascular responses ( Fig. 1c ). FeTPPS and UA also prevented Aβ-induced vascular 3-NT formation ( Fig. 1b ). UA and L-NNA did not attenuate Aβ-induced ROS formation ( Supplementary Fig. 2 ), indicating that the suppression of nitration by these agents was not due to ROS scavenging. Thus, peroxynitrite formation in cerebral blood vessels is needed for the cerebrovascular effects of Aβ. 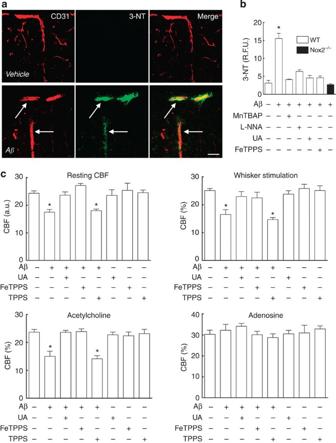Figure 1: Vascular nitrosative stress mediates the vasomotor dysfunction induced by Aβ. 3-NT immunoreactivity, a marker of peroxynitrite, induced by neocortical superfusion of Aβ1–40(Aβ, 5 μM) increases in CD31-positive penetrating arterioles in the somatosensory cortex (arrows;a). The nitration is suppressed by local application of the free radical scavenger MnTBAP, the NOS inhibitor L-NNA, the peroxynitrite scavenger UA or the peroxynitrite decomposition catalyst FeTPPS, and in mice lacking the Nox2 subunit of NADPH oxidase (b). Neocortical superfusion of Aβ1–40attenuates resting CBF and the increase in CBF induced by whisker stimulation or acetylcholine, but not by adenosine. The attenuation is prevented by treatment of UA or FeTPPS, but not its inactive version TPPS (c). Data are presented as mean±s.e.m. *P<0.05 from control, analysis of variance and Tukey’s test;N=5 per group. Figure 1: Vascular nitrosative stress mediates the vasomotor dysfunction induced by Aβ. 3-NT immunoreactivity, a marker of peroxynitrite, induced by neocortical superfusion of Aβ 1–40 (Aβ, 5 μM) increases in CD31-positive penetrating arterioles in the somatosensory cortex (arrows; a ). The nitration is suppressed by local application of the free radical scavenger MnTBAP, the NOS inhibitor L-NNA, the peroxynitrite scavenger UA or the peroxynitrite decomposition catalyst FeTPPS, and in mice lacking the Nox2 subunit of NADPH oxidase ( b ). Neocortical superfusion of Aβ 1–40 attenuates resting CBF and the increase in CBF induced by whisker stimulation or acetylcholine, but not by adenosine. The attenuation is prevented by treatment of UA or FeTPPS, but not its inactive version TPPS ( c ). Data are presented as mean±s.e.m. * P <0.05 from control, analysis of variance and Tukey’s test; N =5 per group. Full size image The microvascular effects of Aβ require PARP/PARG activity Since nitrosative stress activates PARP [31] , [32] , we investigated whether PARP is involved in the neurovascular effects of Aβ. Neocortical application of the PARP inhibitor PJ34 reversed the cerebrovascular alterations induced by Aβ ( Fig. 2a–c ; Supplementary Fig. 1B ). Furthermore, Aβ superfusion did not alter cerebrovascular reactivity in PARP-1 null mice ( Fig. 2 ). Next, we examined whether PARP is also involved in the neurovascular alterations observed in transgenic mice overexpressing APP (tg2576) [22] , [24] , [25] . Superfusion of PJ34 attenuated PARP activity in the underlying neocortex and ameliorated the cerebrovascular dysfunction ( Fig. 3a,b ). Superfusion of the PARG inhibitor adenosine 5′-diphosphate (Hydroxymethyl)pyrrolidinediol, NH 4 (ADP-DPH) also counteracted the cerebrovascular dysfunction both in wild-type (WT) mice with Aβ superfusion and in tg2576 mice ( Figs 2 and 3 ). These findings, collectively, implicate the activity of the PARP/PARG pathway in the mechanisms of neurovascular alterations induced by Aβ. 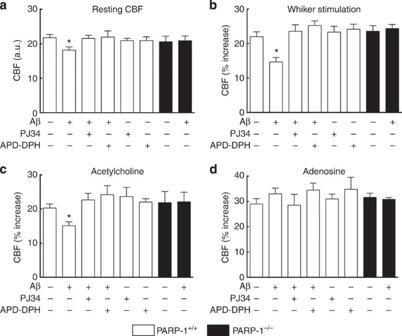Figure 2: PARP/PARG activity is required for the vascular effects of Aβ1–40. Neocortical superfusion of Aβ1–40(Aβ) attenuates resting CBF (a), and the CBF increase evoked by whisker stimulation (b) or acetylcholine (c) in PARP-1+/+mice. The response to adenosine is not affected (d). The vascular effects of Aβ1–40are reversed by neocortical application of the PARP inhibitor PJ34 or the PARG inhibitor APD-DPH, and are not observed in PARP-1−/−mice. Data are presented as mean±s.e.m. a.u., arbitrary unit; *P<0.05, analysis of variance and Tukey’s test;N=5 per group. Figure 2: PARP/PARG activity is required for the vascular effects of Aβ 1–40 . Neocortical superfusion of Aβ 1–40 (Aβ) attenuates resting CBF ( a ), and the CBF increase evoked by whisker stimulation ( b ) or acetylcholine ( c ) in PARP-1 +/+ mice. The response to adenosine is not affected ( d ). The vascular effects of Aβ 1–40 are reversed by neocortical application of the PARP inhibitor PJ34 or the PARG inhibitor APD-DPH, and are not observed in PARP-1 −/− mice. Data are presented as mean±s.e.m. a.u., arbitrary unit; * P <0.05, analysis of variance and Tukey’s test; N =5 per group. 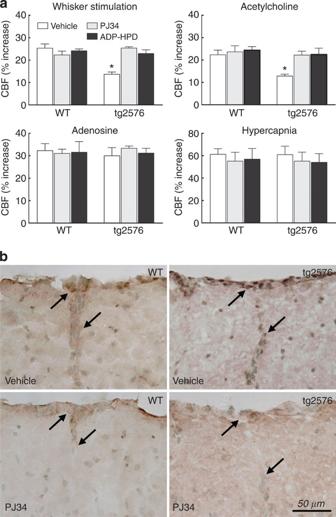Figure 3: PARP and PARG inhibitors reverse the cerebrovascular dysfunction in tg2576 mice. The increase in CBF evoked by whisker stimulation or ACh is attenuated in tg2576 mice, while responses to adenosine and hypercapnia are not affected (a). The cerebrovascular dysfunction is reversed by neocortical application of the PARP inhibitor PJ34 or the PARG inhibitor APD–DPH (a). PJ34 suppresses the increase in PARP activity observed in penetrating pial arterioles of tg2576 mice (arrows). Sections were counterstained with methyl green (b). Data are presented as mean±s.e.m. *P<0.05 from WT vehicle, analysis of variance and Tukey’s test;N=5 per group. Full size image Figure 3: PARP and PARG inhibitors reverse the cerebrovascular dysfunction in tg2576 mice. The increase in CBF evoked by whisker stimulation or ACh is attenuated in tg2576 mice, while responses to adenosine and hypercapnia are not affected ( a ). The cerebrovascular dysfunction is reversed by neocortical application of the PARP inhibitor PJ34 or the PARG inhibitor APD–DPH ( a ). PJ34 suppresses the increase in PARP activity observed in penetrating pial arterioles of tg2576 mice (arrows). Sections were counterstained with methyl green ( b ). Data are presented as mean±s.e.m. * P <0.05 from WT vehicle, analysis of variance and Tukey’s test; N =5 per group. Full size image Aβ induces brain endothelial DNA damage and PARP activation Next, we focused on the cellular mechanisms through which Aβ-induced nitrosative stress leads to PARP activation and endothelial dysfunction. To this end, we first examined whether Aβ-induced nitrosative stress leads to DNA damage and PARP activation. Treatment of brain endothelial cell cultures with Aβ (300 nM), but not its scrambled version, increased the DNA damage marker phospho-γH2A.X, PARP activity and the formation of the PARP reaction product PAR ( Fig. 4 ; Supplementary Fig. 3 ). The phospho-γH2A.X immunoreactivity appeared as nuclear puncta reflecting the sites of DNA damage, whereas the PARP activity signal was more diffuse ( Fig. 4 ), suggesting a broader distribution of PARP reaction products. These effects of Aβ were abolished by ROS scavengers (tempol, MnTBAP), NADPH oxidase inhibition (gp91ds-tat), NOS inhibition (L-NNA) and by the peroxynitrite decomposition catalyst FeTPPS or PARP inhibition (PJ34; Fig. 4c–e ). Thus, Aβ leads to endothelial DNA damage and PARP activation via oxidative–nitrosative stress. 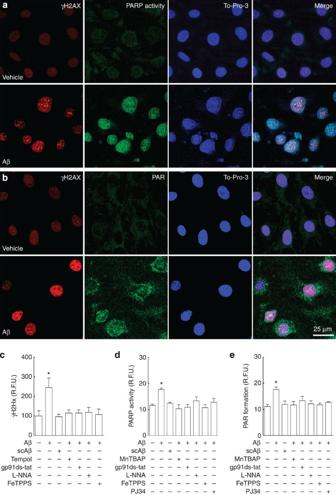Figure 4: Aβ1–40induces DNA damage causing PARP activation and PAR formation in brain endothelial cells. In brain endothelial cell cultures, Aβ1–40(Aβ; 300 nM), but not scrambled Aβ1–40(scAβ), increasesϒH2AX fluorescence, a marker of DNA damage (a–c), PARP activity (a,b,d) and PAR formation (a,b,e). The increases are dampened by the ROS scavengers Tempol and MnTBAP, the NADPH oxidase peptide inhibitor gp91ds-tat, the NOS inhibitor L-NNA and the peroxynitrite decomposition catalyst FeTPPS (c–e). PARP activity (d) and PAR formation (e) are also attenuated by the PARP inhibitor PJ34. To-Pro-3 is a marker of cell nuclei. Data are presented as mean±s.e.m. *P<0.05; analysis of variance and Tukey’s test;N=30–40 cells per group. Figure 4: Aβ 1–40 induces DNA damage causing PARP activation and PAR formation in brain endothelial cells. In brain endothelial cell cultures, Aβ 1–40 (Aβ; 300 nM), but not scrambled Aβ 1–40 (scAβ), increases ϒ H2AX fluorescence, a marker of DNA damage ( a – c ), PARP activity ( a , b , d ) and PAR formation ( a , b , e ). The increases are dampened by the ROS scavengers Tempol and MnTBAP, the NADPH oxidase peptide inhibitor gp91ds-tat, the NOS inhibitor L-NNA and the peroxynitrite decomposition catalyst FeTPPS ( c – e ). PARP activity ( d ) and PAR formation ( e ) are also attenuated by the PARP inhibitor PJ34. To-Pro-3 is a marker of cell nuclei. Data are presented as mean±s.e.m. * P <0.05; analysis of variance and Tukey’s test; N =30–40 cells per group. Full size image Aβ triggers endothelial TRPM2 currents and Ca 2+ increases PAR produced by PARP activity is cleaved to ADPR by PARG [33] . Since ADPR is a potent activator of TRPM2 channels [34] , we examined whether Aβ opens the channels through this mechanism. Abundant TRPM2 immunoreactivity was observed in brain endothelial cells ( Fig. 5a ; Supplementary Fig. 4 ). Aβ, as well as ADPR, injected intracellularly through the patch pipette, induced inward currents blocked by the TRPM2 antagonists N-(p-Amylcinnamoyl)anthranilic acid (ACA) and 2-Aminoethoxydiphenyl borate (2-APB), or by TRPM2 knockdown using short interfering RNA (siRNA; Fig. 5b–d ; Supplementary Fig. 5 ). Analysis of current–voltage relationships demonstrated the conductance characteristics of TRPM2 channels ( Fig. 5b ) [28] , [35] . Consistent with an involvement of NADPH oxidase-derived ROS, NO and peroxynitrite, Aβ-induced TRPM2 currents were blocked by MnTBAP, gp91ds-tat and L-NNA ( Fig. 5d ). In addition, Aβ-induced currents were attenuated by PJ34 and by the PARG inhibitor ADP-HPD, pointing to an involvement of PARP and PARG ( Fig. 5d ). ADPR currents were not attenuated by these antagonists ( Fig. 5d ), ruling out a direct effect of these drugs on the channel. Since activation of TRPM2 leads to massive increases in Ca 2+ into the cells and endothelial cell dysfunction [28] , [29] , [35] , we tested whether Aβ increases intracellular Ca 2+ through TRPM2 channels. Aβ increased intracellular Ca 2+ , an effect attenuated by pretreatment with 2-APB or ACA, and by TRPM2 knockdown ( Fig. 6 ). The effect was dependent on extracellular Ca 2+ and was larger than that produced by the well-established TRPM2 activator H 2 O 2 at concentrations of 0.5–1 mM ( Supplementary Figs 6 and 7 ). These observations, collectively, indicate that Aβ induces TRPM2 currents in endothelial cells, which are mediated by PARP and PARG activity and lead to large and sustained increases in intracellular Ca 2+ . 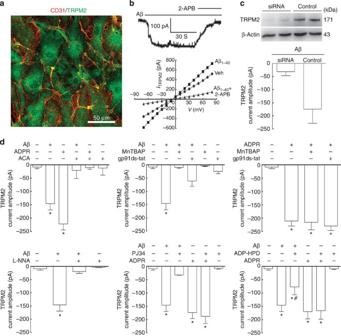Figure 5: Aβ1–40activates sustained TRPM2 currents in brain endothelial cells. TRPM2 is expressed in CD31-positive brain endothelial cell cultures (bEnd.3 cells; seeSupplementary Fig. 4for the specificity of the immunostain) (a). Aβ1–40(Aβ) and the channel activator ADPR induce inward currents with the conductance characteristics of TRPM2 currents (b). The currents are blocked by the TRPM2 inhibitor 2-APB or 2-ACA, or TRPM2 knockdown (b–d). Aβ-induced TRPM2 currents are antagonized by the ROS scavenger MnTBAP, the NADPH oxidase peptide inhibitor gp91ds-tat, the NOS inhibitor L-NNA, the PARP inhibitor PJ34 and the PARG inhibitor ADP-HPD. ADPR-induced TRPM2 currents are unaffected by these antagonists. Data are presented as mean±s.e.m. *P<0.05;#P<0.05 from Aβ1–40-induced currents; analysis of variance and Tukey’s test;N=4–24 cells per group. Figure 5: Aβ 1–40 activates sustained TRPM2 currents in brain endothelial cells. TRPM2 is expressed in CD31-positive brain endothelial cell cultures (bEnd.3 cells; see Supplementary Fig. 4 for the specificity of the immunostain) ( a ). Aβ 1–40 (Aβ) and the channel activator ADPR induce inward currents with the conductance characteristics of TRPM2 currents ( b ). The currents are blocked by the TRPM2 inhibitor 2-APB or 2-ACA, or TRPM2 knockdown ( b – d ). Aβ-induced TRPM2 currents are antagonized by the ROS scavenger MnTBAP, the NADPH oxidase peptide inhibitor gp91ds-tat, the NOS inhibitor L-NNA, the PARP inhibitor PJ34 and the PARG inhibitor ADP-HPD. ADPR-induced TRPM2 currents are unaffected by these antagonists. Data are presented as mean±s.e.m. * P <0.05; # P <0.05 from Aβ 1–40 -induced currents; analysis of variance and Tukey’s test; N =4–24 cells per group. 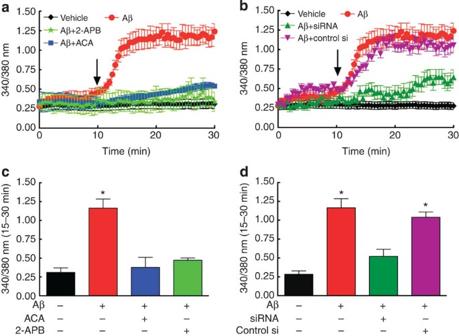Figure 6: Aβ1–40induces large and sustained increases in intracellular Ca2+via TRPM2 channels in brain endothelial cells. The Aβ1–40(Aβ)-induced increases in intracellular Ca2are attenuated by the mechanistically distinct TRPM2 inhibitors 2-APB and ACA (a,c) or by TRPM2 knockdown using siRNA, but not control siRNA (control si) (b,d). Data are presented as mean±s.e.m. *P<0.05; analysis of variance and Tukey’s test;N=6–10 per group. Full size image Figure 6: Aβ 1–40 induces large and sustained increases in intracellular Ca 2+ via TRPM2 channels in brain endothelial cells. The Aβ 1–40 (Aβ)-induced increases in intracellular Ca 2 are attenuated by the mechanistically distinct TRPM2 inhibitors 2-APB and ACA ( a , c ) or by TRPM2 knockdown using siRNA, but not control siRNA (control si) ( b , d ). Data are presented as mean±s.e.m. * P <0.05; analysis of variance and Tukey’s test; N =6–10 per group. Full size image TRPM2 contributes to Aβ-induced neurovascular dysfunction To investigate the potential involvement of TRPM2 channels in vivo , we examined the effect of neocortical application of 2-APB or ACA on the endothelial dysfunction induced by Aβ. These TRPM2 inhibitors did not affect resting cerebrovascular responses but prevented the cerebrovascular effects of Aβ in WT mice and reversed the cerebrovascular dysfunction observed in tg2576 mice ( Fig. 7 ). Similarly, the cerebrovascular dysfunction was not observed in TRPM2-null mice ( Fig. 8 ), providing nonpharmacological evidence for a critical involvement of these channels in the neurovascular and endothelial alterations induced by the Aβ peptide also in vivo . 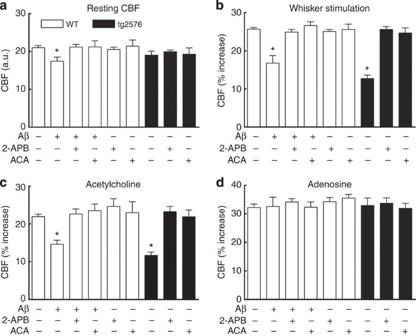Figure 7: TRPM2 inhibition rescues the endothelial dysfunction induced by Aβ1–40in vivo. Neocortical application of 2-APB or ACA has no effect on resting CBF (a), but it prevents the reduction in resting CBF induced by neocortical superfusion of Aβ1–40(Aβ) (a). 2-APB or ACA also rescues the attenuation in the CBF increase evoked by whisker stimulation (b) or acetylcholine (c) induced by Aβ1–40or observed in tg2576 mice. The CBF increase induced by adenosine is unaffected (d). Data are presented as mean±s.e.m. *P<0.05; analysis of variance and Tukey’s test;N=5–6 per group. Figure 7: TRPM2 inhibition rescues the endothelial dysfunction induced by Aβ 1–40 in vivo . Neocortical application of 2-APB or ACA has no effect on resting CBF ( a ), but it prevents the reduction in resting CBF induced by neocortical superfusion of Aβ 1–40 (Aβ) ( a ). 2-APB or ACA also rescues the attenuation in the CBF increase evoked by whisker stimulation ( b ) or acetylcholine ( c ) induced by Aβ 1–40 or observed in tg2576 mice. The CBF increase induced by adenosine is unaffected ( d ). Data are presented as mean±s.e.m. * P <0.05; analysis of variance and Tukey’s test; N =5–6 per group. 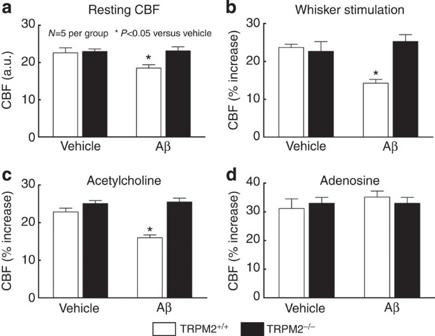Figure 8: Aβ1–40-induced neurovascular dysfunction is not observed in TRPM2-null mice. Neocortical superfusion of Aβ1–40(Aβ) does not attenuate resting CBF (a), or the increase in CBF induced by whisker stimulation (b) or acetylcholine (c) in TRPM2-null mice. Responses to adenosine were not altered (d). Data are presented as mean±s.e.m. *P<0.05; analysis of variance and Tukey’s test;N=5 per group. Full size image Figure 8: Aβ 1–40 -induced neurovascular dysfunction is not observed in TRPM2-null mice. Neocortical superfusion of Aβ 1–40 (Aβ) does not attenuate resting CBF ( a ), or the increase in CBF induced by whisker stimulation ( b ) or acetylcholine ( c ) in TRPM2-null mice. Responses to adenosine were not altered ( d ). Data are presented as mean±s.e.m. * P <0.05; analysis of variance and Tukey’s test; N =5 per group. Full size image We used in vivo and in vitro approaches to investigate the downstream mechanisms of the cerebrovascular dysfunction induced by Aβ. Several new findings were obtained. First, we provided evidence for a critical role of peroxynitrite in the mechanisms of the dysfunction. Second, we found that PARP activity is required for the cerebrovascular effects of Aβ, both in a neocortical application model and in APP-overexpressing mice. Third, we established that Aβ rapidly induces DNA damage, PARP activation and PAR formation in endothelial cells, effects triggered by oxidative–nitrosative stress. Fourth, we demonstrated that Aβ activates a typical TRPM2 channel conductance in endothelial cells leading to intracellular Ca 2+ overload. Fifth, we provided evidence that such TRPM2 activation depends on oxidative–nitrosative stress and requires PARP and PARG activity. Sixth, we demonstrated that TRPM2 channels are also involved in the deleterious effects of Aβ on endothelial function in vivo . These novel observations, collectively, implicate, for the first time, PARP and TRPM2 channels in the endothelial and neurovascular dysfunction induced by Aβ and provide evidence for a previously unappreciated mechanism by which Aβ-induced oxidative–nitrosative stress alters cerebrovascular regulation in models of AD. We found that the peroxynitrite scavenger FeTPPS and UA prevent the vascular nitration and counteract the cerebrovascular dysfunction in full. These agents did not affect vascular ROS production, ruling out that their effects on nitration and CBF regulation were secondary to suppression of oxidative stress. Although it was already established that Aβ induces nitrosative stress in cerebral arterioles [19] , [31] , it was not known whether peroxynitrite contributes to the dysfunction and, if so, through which mechanisms. Since peroxynitrite induces DNA double-strand breaks [32] , [33] , [36] , we explored whether activation of the DNA repair enzyme PARP was involved in the dysfunction. We found that PARP inhibition completely reverses the deleterious vascular effects of exogenous Aβ, and that Aβ does not disrupt cerebrovascular function in PARP-1-null mice. Furthermore, PARP inhibition fully reversed the vascular impairment observed in tg2576 mice. These findings, collectively, provide evidence that Aβ-induced peroxynitrite formation and subsequent PARP activation are critical factors, downstream of ROS, responsible for the cerebrovascular dysfunction. Having established that PARP activity is needed for the alterations in vascular regulation in vivo , we used endothelial cell cultures to investigate the cellular mechanisms of the effect. As suggested by the results in vivo , Aβ produced DNA damage, PARP activation and PAR formation in endothelial cultures. PARP activation in energy-starved tissue has been thought to contribute to cell dysfunction and death by exacerbating energy depletion related to futile regeneration of NAD [32] , [33] , [36] . However, considering the pleiotropic actions of PARP, which also includes proinflammatory and death-promoting effects [37] , the specific contribution of PARP activity to energy depletion and whether the magnitude of the depletion is sufficient to induce cell dysfunction remains unclear [38] . On the other hand, PARP activity generates PAR, which is cleaved to ADPR by PARG [39] , [40] . In turn, ADPR activates TRPM2 channels leading to excessive influx of Ca 2+ and other ions that could alter endothelial function [26] , [28] , [41] , [42] . Therefore, we tested the novel hypothesis that the effects of Aβ on endothelial function are mediated by PARP activity-induced activation of TRPM2 channels. To this end, we first established that Aβ increases PARP activity and PAR production in endothelial cells, and that this effect is associated with DNA damage and requires NADPH-derived ROS, NO and peroxynitrite. Then, we used whole-cell patch clamping to investigate the effect of Aβ on endothelial TRPM2 channel activity. We found that Aβ induces an inward current with the electrophysiological characteristics of TRPM2 currents, which is abolished by TRPM2 inhibition or by TRPM2 knockdown using siRNA. Consistent with an involvement of peroxynitrite, PARP and PARG, TRPM2 currents were suppressed by inhibition of NO or ROS production, and by PARP and PARG inhibitors. Importantly, the current induced by the TRPM2 activator ADPR [27] , [28] , delivered intracellularly through the patch pipette, was not affected by ROS scavengers or PARP and PARG inhibitors, ruling out direct effects of these pharmacological agents on the channel. Since endothelial TRPM2 channels are also activated by oxidative stress [28] , Aβ-induced ROS could activate TRPM2 channels directly. However, this is unlikely because PARP inhibition blocks Aβ-induced TRPM2 currents. Furthermore, PARP inhibition does not affect the ROS production triggered by Aβ, attesting to the fact that PARP activity is downstream of ROS in the signalling events leading to TRPM2 activation. The fact the TRPM2 currents triggered by Aβ are suppressed by inhibition of PARP or PARG also rules out direct effects of Aβ on TRPM2 channels. We found that TRPM2 channel inhibitors prevent the endothelial dysfunction induced by exogenous Aβ and reverse such dysfunction in tg2576 mice. Similarly, Aβ did not alter endothelial function in TRPM2-null mice, providing nonpharmacological evidence of involvement of TRPM2 in the cerebrovascular effects of the peptide. These findings provide evidence that the TRPM2 channel activation observed in endothelial cultures is reflected in disturbances of endothelial cell regulation in vivo . Since some of the effects of TRPM2 channels are sex-specific [43] , it would be of interest to investigate whether there are differences in the involvement of these channels in Aβ-induced vascular dysfunction in male and female mice. Interestingly, TRPM2 inhibition or genetic deletion not only improved endothelial-dependent responses but also restored the increase in CBF induced by neural activity. This finding is not surprising considering the emerging role of endothelial cells in the full expression of the increase in CBF evoked by neural activity [44] . The mechanisms by which TRPM2 channels contribute to neurovascular coupling dysfunction remain to be established. In addition to vascular cells, involvement of TRPM2 on brain cells cannot be ruled out. Irrespective of the effect on functional hyperaemia, however, the in vivo findings corroborate the in vitro evidence linking Aβ to TRPM2 activation and suggest for the first time an involvement of TRPM2 in the endothelial vasomotor dysfunction induced by Aβ. Our data, collectively, suggest the following hypothetical sequence of events in the endothelial dysfunction induced by Aβ ( Fig. 9 ). Activation of innate immunity receptors, that is, CD36 (ref. 21 ) or RAGE [45] , by Aβ leads to production of the ROS superoxide by NADPH oxidase. Superoxide reacts with NO derived from eNOS baseline activity in endothelial cells to form PN, which, in turn, induces DNA damage resulting in PARP activation and PAR formation. ADPR, generated by PARG cleavage of PAR, may then interact with the Nudix domain of TRPM2 opening the channel. However, how does TRPM2 channel activity lead to endothelial dysfunction? We found that the activation of TRPM2 channels by Aβ induces large and sustained increases in endothelial Ca 2+ . Similar Ca 2+ increases were previously observed with H 2 O 2 -dependent activation of endothelial TRPM2 channels, leading to increases in endothelial permeability or apoptosis [28] , [29] . Furthermore, in microglia TRPM2 activation triggers sustained elevations in intracellular Ca 2+ leading to signalling dysfunction [46] , [47] . Other ions, such as Na + , entering the cells through TRPM2 channels could also participate in the dysfunction [26] . It is therefore likely that the mechanisms by which Aβ-induced oxidative–nitrosative stress interferes with endothelial function involve TRPM2-dependent alterations in ionic homeostasis, resulting in suppression of endothelium-dependent vasoactivity. However, the elucidation of the specific pathways involved in the dysfunction downstream of Ca 2+ will require additional investigations. 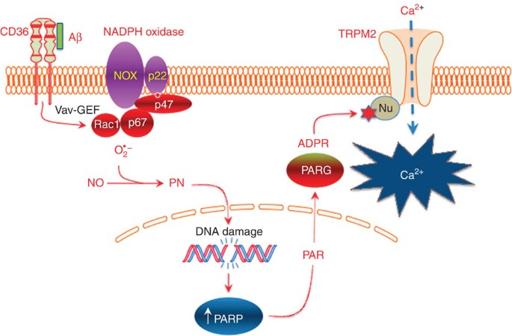Figure 9: Presumed signalling pathways through which Aβ1–40activates endothelial TRPM2 channels. Aβ1–40(Aβ) activates the innate immunity receptor CD36 leading to production of superoxide via NADPH oxidase. Superoxide reacts with NO, made continuously in endothelial cells, to form peroxynitrite (PN). PN induces DNA damage, which, in turn, activates PARP. ADPR formation by PARG cleavage of PAR activates the Nudix (Nu) domain of TRPM2 leading to massive increases in intracellular Ca2+, which induce endothelial dysfunction. However, the involvement of other TRPM2-permeable anions, such as Na+, cannot be ruled out. In a multicellular context, for example,in vivo, PN, a diffusible agent, could also be produced by other vascular cells, and diffuse into endothelial cells to activate this pathway. Figure 9: Presumed signalling pathways through which Aβ 1–40 activates endothelial TRPM2 channels. Aβ 1–40 (Aβ) activates the innate immunity receptor CD36 leading to production of superoxide via NADPH oxidase. Superoxide reacts with NO, made continuously in endothelial cells, to form peroxynitrite (PN). PN induces DNA damage, which, in turn, activates PARP. ADPR formation by PARG cleavage of PAR activates the Nudix (Nu) domain of TRPM2 leading to massive increases in intracellular Ca 2+ , which induce endothelial dysfunction. However, the involvement of other TRPM2-permeable anions, such as Na + , cannot be ruled out. In a multicellular context, for example, in vivo , PN, a diffusible agent, could also be produced by other vascular cells, and diffuse into endothelial cells to activate this pathway. Full size image Increasing evidence indicates that AD is a multifactorial disease with multiple pathogenic components [48] , among which, vascular factors play a prominent role [4] , [5] . Not only soluble and oligomeric Aβ impair cerebrovascular function [4] , [5] , but Aβ deposits in cerebral blood vessels (cerebral amyloid angiopathy) are present in virtually all patients with advanced AD, and are extremely harmful to cerebral arterioles [5] , [22] . These deleterious cerebrovascular effects may contribute to the cognitive deficits by reducing cerebral perfusion and promoting ischaemic brain injury [49] , [50] , [51] . Furthermore, impairment of cerebrovascular vasomotor reactivity may accelerate brain Aβ accumulation by preventing its perivascular and transvascular clearance [4] . Therefore, it has become imperative to elucidate the mechanisms by which Aβ alters vascular function and, based on these mechanisms, to develop new therapeutic approaches. DNA damage and PARP activation, in the long run, may also promote irreversible structural damage to cerebral vessels [4] , [5] , [52] by inducing endothelial cell apoptosis through well-established caspase-independent pathways involving AIF [53] . Our data indicate that TRPM2 may be an attractive therapeutic target for the harmful vascular effects of Aβ. TRP inhibitors are being developed for several neuropsychiatric diseases [54] and their use in AD patients may help to counteract the vascular component of the pathogenic process. In conclusion, we have demonstrated that the cerebrovascular dysfunction induced by exogenous Aβ or in APP mice requires PARP activity triggered by oxidative–nitrosative stress. The dysfunction depends on activation of TRPM2 channels in cerebral endothelial cells resulting in increases in intracellular Ca 2+ . The findings shed new light on the downstream mechanisms by which Aβ-induced oxidative–nitrosative stress leads to cerebrovascular dysfunction and raises the possibility that endothelial TRPM2 channels are a putative therapeutic target to counteract the deleterious cerebrovascular effects of Aβ. Mice All procedures were approved by the Institutional Animal Care and Use Committee of Weill Cornell Medical College. Experiments were conducted in C57BL/6J mice (The Jackson Laboratories), in mice lacking PARP-1 (The Jackson Laboratories) or Nox2, bred on a C56BL/6J background [55] , [56] , and in transgenic mice overexpressing the Swedish mutation of APP (tg2576) [17] . TRPM2-null mice [57] and WT controls were generously provided by Drs Herson and Traystman. All mice were male and 3- to 4-month-old. Age-matched nontransgenic littermates served as controls. Mice were randomly assigned to the experimental groups and experiments were performed in a blinded manner. General surgical procedures and CBF monitoring As described in detail previously, mice were anaesthetised with isoflurane (1–2%), followed by urethane (750 mg kg −1 ; intraperitoneally (i.p.)) and α-chloralose (50 mg kg −1 ; i.p.). A femoral artery was cannulated for recording of arterial pressure and monitoring of blood gasses. Rectal temperature was monitored and controlled. For CBF monitoring, a small opening was drilled in the parietal bone, the dura was removed and the site was superfused with a modified Ringer solution (37 °C; pH 7.3–7.4) [17] , [18] , [21] , [22] , [24] , [25] . Relative CBF was continuously monitored at the site of superfusion with a laser-Doppler flow probe (Vasamedic). Experimental protocol for CBF experiments CBF recordings were started after arterial pressure and blood gases were in a steady state ( Supplementary Tables 1–5 ). All pharmacological agents studied were dissolved in Ringer’s solution, unless otherwise indicated. To study the increase in CBF produced by somatosensory activation, the whiskers were activated by side-to-side deflection for 60 s. The endothelium-dependent vasodilators acetylcholine (10 μM; Sigma) was topically superfused for 3–5 min, and the resulting change in CBF was monitored. CBF responses to the NO donor SNAP (50 μM; Sigma) or the smooth muscle relaxant adenosine (400 μM; Sigma) were also tested [21] , [22] , [24] , [25] . Hypercapnia (PCO 2 to 50–60 mm Hg) was induced by introducing 5% (vol/vol) CO 2 in the circuit of ventilator, and the resulting CBF increase was recorded [22] . CBF responses were tested before and after neocortical superfusion with Aβ 1–40 (5 μM) for 30–45 min, freshly solubilized in dimethylsulphoxide (DMSO) to avoid subsequent peptide aggregation [18] , [31] . The final concentration of DMSO (<0.2%) had no cerebrovascular effects [31] . The Aβ 1–40 concentrations were selected based on previous dose–response studies [58] . We have previously demonstrated that this model of Aβ 1–40 application alters endothelial function in arterioles in the fields of superfusion and reproduces in full the cerebrovascular dysfunction observed in Tg2576 mice [18] , [58] . In some studies, the effect of Aβ was examined before and 30 min after superfusion with Ringer’s solution containing the peroxynitrite scavenger UA (100 μM; Cayman) [59] , the peroxynitrite decomposition catalyst 5,10,15,20-Tetrakis(4-sulfonatophenyl)porphyrinato Iron (III), Chloride (FeTPPS; 20 μM; EMD Millipore) [59] , its inactive version TPPS (20 μM; EMD Millipore) [59] , the PARP inhibitor PJ34 (3 μM; Sigma) [60] , [61] or the TRPM2 channel inhibitors 2-APB (2-APB; 40 μM; Sigma) or N-(p-Amylcinnamoyl)anthranilic acid (ACA; 20 μM; Sigma). Drugs were tested at concentrations previously established to be relatively selective in this or similar models [59] , [60] , [62] , [63] . 3-NT and CD31 immunohistochemistry As described in detail elsewhere [59] , mice were deeply anaesthetised with 5% isoflurane and perfused transcardiacally with saline. Brains were removed and frozen, and brain sections (thickness: 14 μm) were cut through the somatosensory cortex underlying the cranial window (0.38 to −1.94 mm from Bregma) using a cryostat and collected at 100-μm intervals. To assure uniformity of the immunolabel, sections from controls and treatment groups were processed at the same time and under the same condition. Sections were fixed in ethanol and incubated with rabbit anti-mouse 3-NT (1:200; EMD Millipore) followed by a fluorescein isothiocyanate (FITC) goat anti-rabbit secondary antibody (1:200; Molecular Probes). For simultaneous visualization of 3-NT and the endothelial marker CD31, sections were incubated with a rat anti-mouse CD31 monoclonal antibody (1:100; BD Biosciences), followed by a Texas Red goat anti-rat secondary antibody (1:200; Molecular probes). The specificity of the immunolabel was tested by processing sections without the primary antibody or after pre-adsorption with the antigen [59] . The specificity of the 3-NT immunostain was assessed as previously described [64] . Brain sections were examined with a fluorescence microscope (Eclipse E800; Nikon) equipped with Texas Red and FITC filter sets. Images were acquired with a computer-controlled digital monochrome camera (Coolsnap; Robert Scientific) using the same fluorescence settings. Cerebrovascular 3-NT immunoreactivity in the different conditions studied ( n =5 per group) was quantified using the IPLab software (Scanalytics). After background subtraction of the camera dark current, pixel intensities of 3-NT fluorescent signal over CD31-positive vessels were quantified. Ten randomly selected somatosensory cortex sections per mouse were studied. For each section, fluorescence intensities were divided by the total number of pixels, averaged and expressed as relative fluorescence units. ROS detection in vivo As described in detail elsewhere [21] , [24] , dihydroethidine (Molecular Probes; 2 μM) was superfused on the somatosensory cortex for 60 min. In some experiments, dihydroethidine was co-applied with UA (100 μM; Calbiochem) or the NOS inhibitor L-NNA (1 mM; Cayman). At the end of the superfusion period, the brain was removed, sectioned (thickness: 20 μm) and processed for detection of ROS-dependent fluorescence as previously described [21] , [24] . Detection of PARP enzymatic activity in vivo PARP enzymatic activity was detected using a histochemical method adapted from ref. 65 . Mice were perfused transcardiacally with heparinized saline (1,000 U ml −1 ), their brains were removed and the region underlying the cranial window was sectioned (16 μm) using a cryostat. Sections were fixed for 10 min in 95% ethanol at −20 °C, permeabilized by 0.1% Triton X-100 in 100 mM Tris, pH 8.0, for 15 min and then incubated with a reaction mixture, containing 10 mM MgCl 2 , 1 mM dithiothreitol, 30 μm biotinylated NAD + in 100 mM Tris (pH 8.0), for 30 min at 37 °C. After washing in PBS, the sections were treated with peroxidase-conjugated streptavidin (1:100) for 30 min, visualized with a DAB substrate kit (Vector Laboratories, Burlingame, CA, USA), counterstained with Methyl Green and examined under a light microscope (Nikon Eclipse 80i). The specificity of the stain was established using the following: (a) brain sections from PARP-1 null mice, (b) WT mice superfused with the PARP inhibitor PJ34 (30 μM) and (c) sections incubated with a biotinylated NAD + -free reaction mixture. Brain sections from mice superfused with bleomycin (200 μg ml −1 , Sigma), an agents that induces DNA strand breaks, served as positive control. Brain endothelial cell cultures and immunocytochemistry Mouse brain endothelial cells (bEND.3 cells; American Type Culture Collection) were cultured to confluence on coverslips and exposed to Aβ 1–40 (300 nM; rPeptide) or scrambled Aβ 1–40 (300 nM; rPeptide) for 30 min. This concentration was used because it is comparable to that achieved in the brain of AD patients [66] . In some studies, cultures were pretreated for 30 min with vehicle or with the ROS scavenger Tempol (1 mM; Sigma) or MnTBAP (30 μM; EMD Millipore), the NOX2 peptide inhibitor gp91ds-tat (1 μM), L-NNA (10 μM), FeTPPS (20 μM) or PJ34 (30 μM). For TRPM2 immunocytochemistry, cells were fixed in 4% (wt/vol) PFA, washed and processed for double labelling of TRPM2 (1:200; anti-rabbit; Alomone) and CD31 (1:200; anti-rat; BD Biosciences). Cells were then washed and incubated with cy5-conjugated anti-rat IgG (CD31) and FITC-conjugated anti-rabbit IgG (TRPM2) secondary antibodies (Jackson ImmunoResearch). The specificity of the labelling was established by omitting the primary antibody or by pre-absorption with the antigen. Images were acquired using a confocal microscope (Leica). DNA damage, PARP activity and PAR in endothelial cells PARP activity was detected as described for the in vivo experiments, except that the reaction product was visualized by FITC-conjugated streptavidin. Cells were fixed for 10 min in 95% ethanol at −20 °C, permeabilized by 0.1% Triton X-100 in 100 mM Tris (pH 8.0) for 15 min and then incubated with a reaction mixture, containing 10 mM MgCl 2 , 1 mM dithiothreitol, 30 μm biotinylated NAD + in 100 mM Tris (pH 8.0), for 30 min at 37 °C. PJ34 (30 μM) or a biotinylated NAD + -free reaction mixture was used as a negative control. Then, cells were incubated with FITC-conjugated streptavidin (1:100; Invitrogen) to detect incorporated biotin signals, a marker of PARP activity. DNA damage was assessed using the phosphorylated histone variant γH2A.X [67] (Ser139; 1:100; anti-rabbit; EMD Millipore). A donkey cyanine dye (Cy)5-conjugated anti-rabbit IgG (1:200; Jackson ImmunoResearch) was used as a secondary antibody. After washing in PBS, cells were counterstained with the nucleic acid marker To-Pro-3 (1:1,000; Invitrogen). Cells were processed under identical conditions and imaged with the confocal microscope using identical settings. To determine Aβ-induced DNA damage and PARP activity, staining intensity of γH2A.X or PARP activity was quantified using ImageJ and expressed in arbitrary units. To assess PAR formation, cells were fixed for 20 min in 4% PFA at 4 °C and permeabilized by 0.1% Triton X-100 in 0.1% sodium citrate (pH 6.0) for 2 min at 4 °C. After blocking with 1% normal donkey serum and washing in PBS, cells were incubated with γH2A.X (Ser139; 1:100; anti-rabbit; EMD Millipore) and PAR antibodies (10 μg ml −1 ; anti-mouse; Enzo) at 4 °C overnight. Then, cells were incubated with donkey FITC-conjugated anti-mouse (1:200; Jackson ImmunoResearch) and Cy5-conjugated anti-rabbit secondary IgGs (1:200; Jackson ImmunoResearch). After washing in PBS, cells were counterstained with the nucleic acid marker To-Pro-3 (1:1,000; Invitrogen). Confocal images were acquired as above. Cells were processed under identical conditions and scanned at the confocal microscope using identical settings. Omission of primary antibody was used as negative control and cells treated with bleomycin (200 μg ml −1 ) served as positive control. To determine Aβ-induced DNA damage and PAR formation, staining intensity of phospho-γH2A.X or PAR was quantified using ImageJ and expressed in relative fluorescence units. TRPM2 currents in endothelial cell cultures TRPM2 channel currents were recorded using whole-cell patch clamp [68] in subconfluent endothelial cell cultures. TRPM2 channel opening was induced with Aβ 1–40 (300 nM) in the bath solution or intracellular injection of ADP ribose (ADPR; 100 μM) [62] , [63] through the patch pipette. TRPM2 currents were recorded at the holding potential (−50 mV); currents were normalized by the cell capacitance. In some experiments, cells were pretreated for 30 min with 2-APB (30 μM), ACA (20 μM), MnTBAP (100 μM), the NOX2 peptide inhibitor gp91ds-tat (1 μM), L-NNA (10 μM), FeTPPS (20 μM), PJ34 (30 μM) or the PARG inhibitor ADP-HPD (2 μM; EMD Millipore). Drugs were used at concentrations previously established to be relatively specific in similar preparations [69] . 2-APB also inhibits store-operated Ca 2+ entry, but at the concentration used is a relatively specific TRPM2 inhibitor [62] , [63] . To complement the results obtained with 2-APB, we also used the mechanistically distinct TRPM2 inhibitor ACA [62] . Similarly, ADP-HPD was used at a concentration relatively specific for PARG inhibition [69] . TRPM2 knockdown in endothelial cell cultures bEnd cells (1 × 10 5 cells in a 35-mm dish) were transfected with TRPM2 siRNA (FlexiTube GeneSolution GS28240, Qiagen) or control siRNA (Qiagen) using oligofectamine 2000 (Invitrogen). The reduction of TRPM2 protein in whole-cell lysates was confirmed with western blot analysis using anti-TRPM2 antibodies (1:200; ant-rabbit; alomone labs). Full scan images of western blots are presented in Supplementary Fig. 8 . TRPM2 currents or intracellular Ca 2+ were assessed 48 h after the transfection. Assessment of cytoplasmic Ca 2+ in endothelial cells Cytosolic-free Ca 2+ was determined using fura-2/AM as indicator (Molecular Probes) in confluent monolayers of endothelial cells grown on poly-L-lysine-coated glass bottom Petri dishes. The bEND.3 cells were loaded with fura-2/AM (5 μM) in artificial cerebral spinal fluid (aCSF) composed of (in mmol l −1 ): 124, NaCl; 26, NaHCO 3 ; 5, KCl; 1, NaH 2 PO 4 ; 2, MgSO 4 ; 2, CaCl 2 ; 10, glucose; 4.5, lactic acid; oxygenated with 95% O 2 and 5% CO 2 , pH 7.4) for 60 min. The cells then were washed three times with aCSF and incubated in aCSF for an additional 15 min at room temperature. The Petri dish was mounted on a Nikon inverted microscope and images were acquired using a fluorite oil-immersion lens (Nikon CF UV-F X40; numeric aperture 1.3). Aβ 1–40 (300 nM) was added directly to the Petri dish. In some experiments, the bEnd.3 cells were pretreated with the TRPM2 inhibitor ACA (20 μM) or 2-APB (30 μM) for 20 min. Fura-2 was alternately excited through narrow band-pass filters (340±7.5 and 380±10 nm). An intensified CCD camera (Retiga ExI) recorded the fluorescence emitted by the indicator (510±40 nm). Fluorescent images were digitized and backgrounds were subtracted. Eight to fourteen endothelial cells were simultaneously recorded in a randomly selected field. At the end of each experiment, cell viability was examined by testing the response to Ca 2+ ionophore 4-bromo-A23187 (Calbiochem, CA, USA). Fluorescence measurements were obtained from cell somata, and 340/380 nm ratios were calculated for each pixel by using a standard formula [70] . Data analysis Cells and mice were randomly assigned to treatment with inhibitors or vehicle. Histological and electrophysiological analyses were performed in a blinded manner. Data are expressed as means±s.e.m. Two-group comparisons were analysed by the two-tailed t -test. Multiple comparisons were evaluated by the analysis of variance and Tukey’s test. Differences were considered statistically significant for probability values less than 0.05. How to cite this article: Park, L. et al. The key role of transient receptor potential melastatin-2 channels in amyloid-β-induced neurovascular dysfunction. Nat. Commun. 5:5318 doi: 10.1038/ncomms6318 (2014).